Male–female communication triggers calcium signatures during fertilization inArabidopsis Cell–cell communication and interaction is critical during fertilization and triggers free cytosolic calcium ([Ca 2+ ] cyto ) as a key signal for egg activation and a polyspermy block in animal oocytes. Fertilization in flowering plants is more complex, involving interaction of a pollen tube with egg adjoining synergid cells, culminating in release of two sperm cells and their fusion with the egg and central cell, respectively. Here, we report the occurrence and role of [Ca 2+ ] cyto signals during the entire double fertilization process in Arabidopsis . [Ca 2+ ] cyto oscillations are initiated in synergid cells after physical contact with the pollen tube apex. In egg and central cells, a short [Ca 2+ ] cyto transient is associated with pollen tube burst and sperm cell arrival. A second extended [Ca 2+ ] cyto transient solely in the egg cell is correlated with successful fertilization. Thus, each female cell type involved in double fertilization displays a characteristic [Ca 2+ ] cyto signature differing by timing and behaviour from [Ca 2+ ] cyto waves reported in mammals. Fertilization in eukaryotes involves species-specific recognition, local interaction, attachment and eventually fusion of two gametic cells of opposite sex. The fertilization process in flowering plants (angiosperms) is especially complex and requires communication between the cells of two haploid gametophytes [1] . The pollen tube comprises the male gametophyte and consists of a vegetative tube cell that carries two immotile sperm cells. The female gametophyte is composed of the two female gametes (egg and central cell) and accessory cells at opposite poles. Two synergid cells adjoining the egg cell are located at the micropylar entry of the ovule, while antipodal cells neighbouring the central cell are found at the chalazal pole. After sperm cell delivery and fusion of two gamete pairs, a process termed as double fertilization, the fertilized central cell develops into the endosperm and the fertilized egg cell gives rise to the embryo. Numerous cell–cell communication events take place during the attraction of the male towards the female gametophyte and their mutual interaction. It was reported that synergid cells are responsible for pollen tube attraction by secreting species-specific chemotactic peptides [2] , [3] , [4] , [5] . Moreover, they recognize arriving pollen tubes involving cell surface receptors [6] , [7] , [8] and control sperm release [9] , [10] . After pollen tube burst, the two sperm cells rapidly reach the cleft between egg and central cell representing the site of gamete interaction and fusion [11] . Sperm cells interact with female gametes and become activated by egg cell-secreted small proteins [12] . The molecular mechanisms by which the male and female gametes recognize each other and the intracellular signalling events that result in synergid cell death, female gamete activation, control of successful plasmogamy and the prevention of multiple sperm fusion (polyspermy) remain to be identified. In animals, calcium plays a key role during fertilization as a secondary messenger of cell–cell interaction events and triggers, for example, the establishment of a fertilization membrane to prevent polyspermy [13] , [14] , [15] . While the role of calcium signalling during double fertilization in flowering plants still remains to be unveiled, it is known that calcium signalling plays a key role in cell–cell recognition, for example, during the innate immune response to pathogens or the establishment of symbiosis [16] , [17] . Calcium has also known functions during the early stages of fertilization, which include promoting pollen tube growth, guidance and eventually the regulation of its burst [18] , [19] , [20] , [21] . Recently, it was also reported that the arrival of the pollen tube causes [Ca 2+ ] cyto oscillations in synergid cells [20] . This observation opened up the question how the pollen tube and the synergid cells interact with each other to trigger these oscillations, whether this occurred through direct contact or through signals that act at a distance. The first evidence that calcium indeed is also involved during gamete fusion was obtained from in vitro fertilization experiments. Gamete fertilization in maize mediated by calcium chloride was shown to occur in a cell-specific manner and leads to a block of polyspermy [22] . More detailed studies have reported that Ca 2+ influx occurred in this in vitro system after egg–sperm fusion and spreads as a wave front from the fusion site towards the whole cell lasting for up to 30 min (refs 23 , 24 , 25 ). The authors further observed that fusion, but not gamete adhesion triggered a transient [Ca 2+ ] cyto rise in fertilized egg cells and found that cell wall material is formed after fusion likely representing a block to polyspermy functionally similar to the fertilization membrane in animals. These data strongly support the notion that calcium signalling may be of similar importance during double fertilization in plants compared with fertilization in animals. However, in vitro investigations are limited as double fertilization mechanisms involve many timely and accurately regulated cellular interactions to guarantee reproductive success. To visualize when and how calcium transients are triggered during the whole double fertilization process in vivo , and to enable studies on the functional role(s) of [Ca 2+ ] cyto changes during fertilization, we used an enhanced genetically encoded fluorescent calcium sensor. This sensor consists of a calcium-binding domain fused to two fluorophores that are spectrally overlapping. Their proximity and orientation depends on the conformation of the binding domain. Calcium binding therefore results in differential Förster Resonance Energy Transfer (FRET) between the donor and acceptor fluorophores. Most widely used in plants are Yellow Cameleon sensors [26] , [27] , [28] , [29] that contain a calmodulin-based calcium-binding domain. It has been argued, however, that due to the high degree of conservation of calmodulin, cellular pathways might interfere with the sensor, and vice versa [30] . This led to the development of the calcium sensor CerTN-L15, a sensor with enhanced folding, increased brightness and a calcium-binding domain based on troponin C, a protein exclusively found in myocytes [31] . Thus, it is unlikely that CerTN-L15 exhibits strong interactions with plant proteins. By using a modified semi- in vivo system [32] and expressing the improved calcium sensor CerTN-L15 from various female gametophyte cell-type-specific promoters, we were able to monitor [Ca 2+ ] cyto signatures by live-cell imaging throughout the whole double fertilization process in the model plant Arabidopsis . We report that direct contact with the pollen tube apex and not its shank region triggers polarized [Ca 2+ ] cyto oscillations in synergids cells. Furthermore, we link sperm cell dynamics at the gamete fusion site to specific Ca 2+ signatures in both egg and central cells. We show that first Ca 2+ transients precede fertilization, indicating that they might be required for early events such as female gamete activation. A second Ca 2+ transient solely in the egg cell appears associated to sperm–egg fusion and might trigger later events such as a block to polyspermy. Sensor based recording of cell-specific calcium changes To monitor [Ca 2+ ] cyto during the whole double fertilization process, we expressed the Ca 2+ sensor CerTN-L15 (ref. 31 ) under control of cell-type-specific promoters in synergid cells ( MYB98 -promoter; AT4G18770 (ref. 33 )), egg cell ( EC1.1 promoter; AT1G76750 (ref. 12 )) and the central cell ( DD65 -promoter; AT3G10890 (ref. 34 )) as indicated ( Fig. 1a ). This sensor is based on the Ca 2+ −binding domain of troponin C and two spectrally overlapping fluorescent molecules cerulean and citrine that act as donor and acceptor for FRET, respectively. As the CerTN-L15 sensor has not been used in plants before, we first validated its functionality in roots expressing the sensor constitutively under control of a 35S promoter, using a microfluidic device that allows imaging under controlled perfusion of roots [35] . Repeated pulsed treatments with a hyperosmotic solution resulted in [Ca 2+ ] cyto signatures with a minor increase in FRET ratio during the treatment-induced root shrinkage and a steep incline of the FRET ratio after wash-out and return to original root length, followed by a gradual return of the FRET ratio to the baseline ( Supplementary Fig. 1 ). This characteristic signature has been observed before using Yellow Cameleon sensors [29] , [36] indicating that CerTN-L15 is functional in plants. 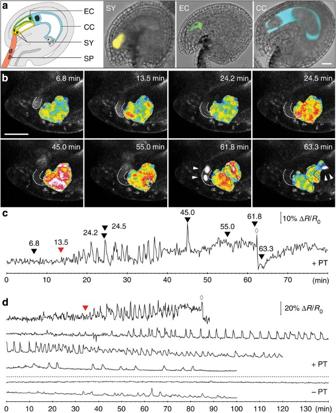Figure 1: [Ca2+]cytosignatures in synergid cells during pollen tube arrival and discharge. (a) Expression of the calcium sensor CerTN-L15 in specific cells of the female gametophyte. Left panel: schematic of an ovule and approaching pollen tube (PT, orange) containing two sperm cells (SP, red) and the vegetative tube nucleus (indicated in blue). The female gametophyte consists of two synergid cells (SY, yellow), one egg cell (EC, green) and one central cell (CC, cyan). Right panels: merged bright field and confocal images of ovules expressing CerTN-L15 in specific cell types (promoters are in parentheses): SY (pMYB98), EC (pEC1) and CC (pDD65). (b) Arrival and discharge of a PT at the SYs. Time series of a PT of the LHR marker line displaying the tube apex (outline of the PT is indicated by dotted lines) approaching SYs (false colour ratiometric images of pMYB98:CerTN-L15). SPs (arrowheads) of this marker line are discharged about 62 min after recording was initiated. The following stages are visible: arrival of a PT (6.8 min), first PT contact with SY (13.5 min), before (24.2 min) and during (24.5 min) an oscillation of [Ca2+]cyto, growth of PT around SY (45.0 min, 55.0 min), PT shortly before (61.8 min) and after (63.3 min) release of SPs. See correspondingSupplementary Movie 1. (c) [Ca2+]cytosignature of SYs. Normalized ratio changes of CerTN-L15 in cells shown inb. Arrowheads indicate time points of images inb. Red arrowhead: first physical contact of PT and SY, diamond: pollen tube burst. (d) Variations of [Ca2+]cytosignatures in SYs. Selection of representative [Ca2+]cytomeasurements in SYs in the presence (+PT, upper panel) or absence of a PT (−PT, lower panel). Note that PT burst occured only in upper example showing high [Ca2]cytoamplitudes. Red arrowhead marks the time point where the first physical contact of a PT and the synergid could be observed, diamond indicates pollen tube burst. The first graph of the lower panel (−PT) shows typical [Ca2+]cytorecording of SY without PT. The second graph displays an exceptional case of spontaneous [Ca2+]cytooscillations in SY without a PT being present. This bahaviour was observed in two out of 13 cases. Scale bars, 20 μm. Figure 1: [Ca 2+ ] cyto signatures in synergid cells during pollen tube arrival and discharge. ( a ) Expression of the calcium sensor CerTN-L15 in specific cells of the female gametophyte. Left panel: schematic of an ovule and approaching pollen tube (PT, orange) containing two sperm cells (SP, red) and the vegetative tube nucleus (indicated in blue). The female gametophyte consists of two synergid cells (SY, yellow), one egg cell (EC, green) and one central cell (CC, cyan). Right panels: merged bright field and confocal images of ovules expressing CerTN-L15 in specific cell types (promoters are in parentheses): SY ( pMYB98 ), EC ( pEC1 ) and CC ( pDD65 ). ( b ) Arrival and discharge of a PT at the SYs. Time series of a PT of the LHR marker line displaying the tube apex (outline of the PT is indicated by dotted lines) approaching SYs (false colour ratiometric images of pMYB98:CerTN-L15). SPs (arrowheads) of this marker line are discharged about 62 min after recording was initiated. The following stages are visible: arrival of a PT (6.8 min), first PT contact with SY (13.5 min), before (24.2 min) and during (24.5 min) an oscillation of [Ca 2+ ] cyto , growth of PT around SY (45.0 min, 55.0 min), PT shortly before (61.8 min) and after (63.3 min) release of SPs. See corresponding Supplementary Movie 1 . ( c ) [Ca 2+ ] cyto signature of SYs. Normalized ratio changes of CerTN-L15 in cells shown in b . Arrowheads indicate time points of images in b . Red arrowhead: first physical contact of PT and SY, diamond: pollen tube burst. ( d ) Variations of [Ca 2+ ] cyto signatures in SYs. Selection of representative [Ca 2+ ] cyto measurements in SYs in the presence (+PT, upper panel) or absence of a PT (−PT, lower panel). Note that PT burst occured only in upper example showing high [Ca 2 ] cyto amplitudes. Red arrowhead marks the time point where the first physical contact of a PT and the synergid could be observed, diamond indicates pollen tube burst. The first graph of the lower panel (−PT) shows typical [Ca 2+ ] cyto recording of SY without PT. The second graph displays an exceptional case of spontaneous [Ca 2+ ] cyto oscillations in SY without a PT being present. This bahaviour was observed in two out of 13 cases. Scale bars, 20 μm. Full size image Pollen tube apex triggers calcium signatures in synergids To record [Ca 2+ ] cyto signatures in cells of the female gametophyte, we performed our measurements on excised Arabidopsis ovules arranged around a pollinated pistil [32] . This semi- in vivo setup was modified to achieve automated time-lapse imaging at high spatiotemporal resolution. When CerTN-L15 was expressed in synergid cells, we observed repeated FRET ratio changes consistent with [Ca 2+ ] cyto increases in 23 out of 25 experiments when the pollen tube successfully interacted with the synergid cells ( Fig. 1b,c ). The [Ca 2+ ] cyto transients occurred with variable periodicity within and among cells with a time interval of 100–200 s and durations of 50–170 s per individual transient. ( Fig. 1d , Supplementary Fig. 2a, Movies 1 and 2 ). Burst of pollen tubes and receptive synergid cell occurred between 30 and 50 min after interaction with synergid cells. [Ca 2+ ] cyto oscillations with low amplitude (lower graphs in Fig. 1d ) did not result in burst. When pollen tubes failed to target the micropyle of the ovule or did not reach the synergid cells, we detected spontaneous weak [Ca 2+ ] cyto fluctuations in two out of 16 trials ( Fig. 1d , lower panel). In both cases, fluctuations were less regular and showed significantly reduced amplitude by comparison with the signatures observed when pollen tubes successfully approached the synergid cells. We conclude from these observations that limited [Ca 2+ ] cyto oscillations can occur spontaneously in synergid cells at a low likelihood. Only pollen tubes that successfully enter the ovule and interact with the synergid cells induce high persistent and effective [Ca 2+ ] cyto oscillations. Consistent with recently published work [37] , we observed that the pollen tube did not burst in the filiform apparatus as suggested previously (reviewed in ref. 37 ). Instead the pollen tube grew for up to 60 min in close proximity and around the synergid cells towards the gamete fusion site before rupture and synergid cell death occurred ( Supplementary Movie 1 ). To investigate whether communication between the pollen tube and the synergid cells occurs already at a distance, or if physical cell–cell contact is required, we monitored the onset of Ca 2+ oscillations as a function of the distance between the two cells. To this end, we visualized the pollen tube apex by developing a novel marker (P LAT52 :RemCA-tagRFP) targeting tagRFP with the carboxyl-terminal (C-terminal) anchor sequence of remorin to the plasma membrane of pollen tubes and introduced it into a homozygous sperm nuclei marker line (P H3.3 :H3.3-mRFP [38] ) resulting in the double marker line LHR (Lat52:tagRFP-T-REM; HTR10:HTR10-mRFP; see Methods for details). In all eight measurements where the onset of [Ca 2+ ] cyto oscillations in synergid cells and the advance of the pollen tube tip could be monitored simultaneously, the first substantial [Ca 2+ ] cyto transients (ratio change >5 σ of baseline of first derivative, see Methods) were detected when the distance between the two cells could no longer be resolved ( Fig. 1b,c ). In three of the 25 experiments, the position of the two synergid cells allowed separate measurements of cytoplasmic CerTN-L15 fluorescence within each cell. We observed that the amplitude and frequency of [Ca 2+ ] cyto oscillations depended on the relative distance and position of the pollen tube tip and either of the two synergid cells. Only the synergid cell in direct contact with the pollen tube tip showed continuous [Ca 2+ ] cyto oscillations ( Fig. 2a,b ). 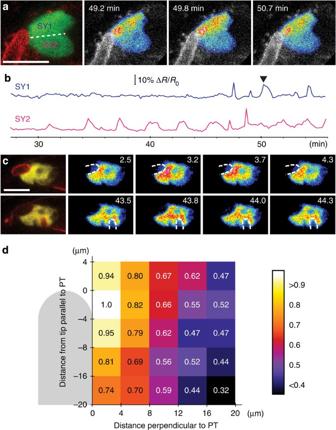Figure 2: [Ca2+]cytosignature in the synergid cell depends on the physical interaction with the pollen tube apex. (a) CerTN-L15 signals observed in each of the two SYs separately. Left panel: merged confocal image of a LHR PT tip (red) in contact with both pMYB98:CerTN-L15 expressing SYs (YFP signal of CerTN-L15 in green). Both SYs can be seen separately (SY1 and SY2). Right panels: one representative [Ca2+]cytotransient (beginning, maximum, end) occurring only in SY1, which is in contact with the PT. LHR pollen is shown in grey scale, ratio changes of CerTN-L15 in SYs are displayed as heat map. (b) Ratio changes recorded for both SYs. The ratio changes of CerTN-L15 were measured in the two SYs separately. Arrowhead marks the [Ca2+]cytotransient shown ina. (c) Local [Ca2+]cytotransients in relation to PT tip position. Two [Ca2+]cytotransients of one time series are shown. [Ca2+]cytotransients with LHR PT tip in contact with the filiform apparatus (upper row) and after being grown around the SYs (lower row). Left panel in both rows: merged confocal image of a LHR PT tip (red) in contact with pMYB98:CerTN-L15 SYs (YFP signal of CerTN-L15 in yellow). Right panels of both rows: time points of corresponding time series before, during and after a transient of [Ca2+]cytoin the SYs (ratio of CerTN-L15 displayed in pseudo colour). The maximum of the [Ca2+]cytois different in both rows and correlates with the position of the PT tip (dotted line indicates the position of the PT according to the signal shown in the left panel). (d) Mapping of amplitudes of [Ca2+]cytotransients in relation to the distance to PT tip. Schematic of a PT tip in contact with a SY. Amplitudes of [Ca2+]cytoelevations were measured in 44 mm regions (indicated as squares) over the SY in time series registered to the PT tip. Measured amplitudes of the maximum number of detected [Ca2+]cytotransients in five independent experiments. Numbers in each square display the normalized average amplitude height. For statistical data, seeSupplementary Fig. 2b. Scale bars, 20 μm. Figure 2: [Ca 2+ ] cyto signature in the synergid cell depends on the physical interaction with the pollen tube apex. ( a ) CerTN-L15 signals observed in each of the two SYs separately. Left panel: merged confocal image of a LHR PT tip (red) in contact with both pMYB98:CerTN-L15 expressing SYs (YFP signal of CerTN-L15 in green). Both SYs can be seen separately (SY1 and SY2). Right panels: one representative [Ca 2+ ] cyto transient (beginning, maximum, end) occurring only in SY1, which is in contact with the PT. LHR pollen is shown in grey scale, ratio changes of CerTN-L15 in SYs are displayed as heat map. ( b ) Ratio changes recorded for both SYs. The ratio changes of CerTN-L15 were measured in the two SYs separately. Arrowhead marks the [Ca 2+ ] cyto transient shown in a . ( c ) Local [Ca 2+ ] cyto transients in relation to PT tip position. Two [Ca 2+ ] cyto transients of one time series are shown. [Ca 2+ ] cyto transients with LHR PT tip in contact with the filiform apparatus (upper row) and after being grown around the SYs (lower row). Left panel in both rows: merged confocal image of a LHR PT tip (red) in contact with pMYB98:CerTN-L15 SYs (YFP signal of CerTN-L15 in yellow). Right panels of both rows: time points of corresponding time series before, during and after a transient of [Ca 2+ ] cyto in the SYs (ratio of CerTN-L15 displayed in pseudo colour). The maximum of the [Ca 2+ ] cyto is different in both rows and correlates with the position of the PT tip (dotted line indicates the position of the PT according to the signal shown in the left panel). ( d ) Mapping of amplitudes of [Ca 2+ ] cyto transients in relation to the distance to PT tip. Schematic of a PT tip in contact with a SY. Amplitudes of [Ca 2+ ] cyto elevations were measured in 44 mm regions (indicated as squares) over the SY in time series registered to the PT tip. Measured amplitudes of the maximum number of detected [Ca 2+ ] cyto transients in five independent experiments. Numbers in each square display the normalized average amplitude height. For statistical data, see Supplementary Fig. 2b . Scale bars, 20 μm. Full size image To support this finding and to investigate whether the synergid [Ca 2+ ] cyto signatures represent global or localized responses, we analysed 78 [Ca 2+ ] cyto peaks and detected the highest amplitude in immediate proximity to the contact site of synergid cell and pollen tube tip ( Fig. 2c ). Progressing pollen tube growth resulted in relocation of the local [Ca 2+ ] cyto maximum that matched the shifted site of contact with the pollen tube tip. To measure whether indeed only the apex or the entire surface of the pollen tube has the capability to elicit a Ca 2+ signature in the synergid cells, we mapped the local amplitudes [Ca 2+ ] cyto peaks ( n =78) in synergid cells in 4 × 4 μm bins across the whole cell. We found that the sensor amplitude gradually decreased with increasing distance from the pollen tube tip ( Fig. 2d , Supplementary Fig. 2b ), consistent with the observation that [Ca 2+ ] cyto is highest at the site where the cells are in direct contact. Moreover, we found that the local sensor amplitude in the synergid cell was the highest in closest proximity to the pollen tube apex and not the shank of the tube ( Fig. 2d , Supplementary Fig. 2b ). Taken together, the separate measurements of neighbouring synergids and the correlation of pollen tube position and localized synergid response demonstrate that physical contact specifically with the pollen tube apex is necessary to induce and maintain [Ca 2+ ] cyto oscillations in the synergid cell. Our measurements in synergid cells further show that there exists not just one excitable zone, but rather large areas of the synergid cell surface are capable of sensing contact with the pollen tube. Sperm cell delivery causes calcium signals in female gametes Once the pollen tube has ruptured and released its content including the two sperm cells, the process of fertilization enters the next stage, the specific interaction and fusion of the two sperm cells with the egg and the central cell, respectively. To investigate whether the interactions between male and female gametes also invoke Ca 2+ transients and whether there is a correlation between calcium signatures and sperm cell movement, we measured [Ca 2+ ] cyto in egg and central cells, separately. When measuring CerTN-L15 signals in the central cell during successful pollen tube rupture ( n =14), we observed a sharp increase in [Ca 2+ ] cyto lasting for approximately 1 min immediately following pollen tube burst and deformation of the central cell in the area of sperm arrival due to explosive release of pollen tube contents ( Fig. 3a,b , t =0 min; Supplementary Movie 3 ). Beyond this short transient, significant [Ca 2+ ] cyto transients were not detectable, independent of fertilization success (see further examples in Supplementary Fig. 3 ). 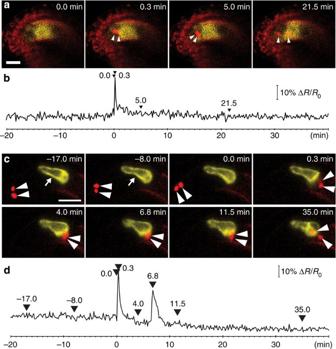Figure 3: [Ca2+]cytosignatures in female gametes during double fertilization. (a) Time series showing arrival of labelled SPs (indicated by arrow heads; LHR marker line) at the gamete fusion site and subsequent plasmogamy with the central cell expressing pDD65:CerTN-L15 (yellow). Images show major steps of the gamete fusion process: directly before PT rupture (0.0 min), after PT rupture and SP arrival (0.3 min), during arrest phase of SPs at the fusion site (5.0 min) and after plasmogamy showing the movement of SP nucleus towards CC nucleus (21.5 min). Scale bar, 20 μm. See alsoSupplementary Movie 3. (b) [Ca2+]cytotransients in the CC during fertilization. Normalized ratio of CerTN-L15 in CC of time series shown ina. Arrowheads indicate time points corresponding to images shown ina. A single ratio change of 27% occurs during SP release (time point 0.3 min). (c) Time series of a LHR pollen fertilizing an ovule expressing pEC1:CerTN-L15 in the egg cell (EC, yellow). From −17.0 to 0.0 min) the PT is in contact with SYs (not visible). SPs (red, marked by arrowheads) release occurred at 0.0 min. Arrest of SPs is visible at the fusion site (4.0 min), movement of one SP nuclei inside egg cytoplasm (6.8–11.5 min) is followed by the separation of SP nuclei (11.5–35 min) indicating fertilization success. Scale bar, 20 μm. See correspondingSupplementary Movie 4. (d) [Ca2+]cytosignals in the EC during fertilization. Normalized ratio changes of CerTN-L15 in the EC of time series shown inc. Arrowheads with time correspond to the images shown inc. Ratio changes can be seen directly after SP release (0.0 min) and during the arrest phase of the SPs at the fusion site (6.8 min) but not after SP separation (11.5–35.0 min). Figure 3: [Ca 2+ ] cyto signatures in female gametes during double fertilization. ( a ) Time series showing arrival of labelled SPs (indicated by arrow heads; LHR marker line) at the gamete fusion site and subsequent plasmogamy with the central cell expressing pDD65:CerTN-L15 (yellow). Images show major steps of the gamete fusion process: directly before PT rupture (0.0 min), after PT rupture and SP arrival (0.3 min), during arrest phase of SPs at the fusion site (5.0 min) and after plasmogamy showing the movement of SP nucleus towards CC nucleus (21.5 min). Scale bar, 20 μm. See also Supplementary Movie 3 . ( b ) [Ca 2+ ] cyto transients in the CC during fertilization. Normalized ratio of CerTN-L15 in CC of time series shown in a . Arrowheads indicate time points corresponding to images shown in a . A single ratio change of 27% occurs during SP release (time point 0.3 min). ( c ) Time series of a LHR pollen fertilizing an ovule expressing pEC1:CerTN-L15 in the egg cell (EC, yellow). From −17.0 to 0.0 min) the PT is in contact with SYs (not visible). SPs (red, marked by arrowheads) release occurred at 0.0 min. Arrest of SPs is visible at the fusion site (4.0 min), movement of one SP nuclei inside egg cytoplasm (6.8–11.5 min) is followed by the separation of SP nuclei (11.5–35 min) indicating fertilization success. Scale bar, 20 μm. See corresponding Supplementary Movie 4 . ( d ) [Ca 2+ ] cyto signals in the EC during fertilization. Normalized ratio changes of CerTN-L15 in the EC of time series shown in c . Arrowheads with time correspond to the images shown in c . Ratio changes can be seen directly after SP release (0.0 min) and during the arrest phase of the SPs at the fusion site (6.8 min) but not after SP separation (11.5–35.0 min). Full size image In the egg cell, we also observed an immediate deformation of its shape that coincided with the pollen tube burst and the rapid delivery of sperm cells ( Fig. 3c ). Analysis of [Ca 2+ ] cyto levels during these events ( n =26) revealed again a sharp increase that coincided with cell deformation and sperm cell arrival ( Fig. 3d , t =0 min). In some experiments, deformation of the egg cell was caused by the growing pollen tube ( Fig. 3c , arrows at time points −17 min and −8 min). However, in these cases, calcium transients were never detected ( Fig. 3d ; Supplementary Figs 4a,b and 6b , Supplementary Movies 4, 5 ). This indicates that mechanical stimulation of the egg cell is not sufficient to cause the detected elevation of [Ca 2+ ] cyto. . While the sharp [Ca 2+ ] cyto peak at t =0 occurred in both female gametes simultaneously during pollen tube burst, an additional extended [Ca 2+ ] cyto transient with more gradual rise and fall times was detected only in the egg cells ( Figs 3d and 4c , Supplementary Figs 3 and 6c ). This second [Ca 2+ ] cyto transient appeared on average 3.8 min (±1.9, n =12) after the pollen tube burst and lasted on average for 3.1 min (±0.66, n =12). The second [Ca 2+ ] cyto transient was detected in all successful fertilization events ( n =10) as shown in Fig. 4c . When fertilization was not successful, the second [Ca 2+ ] cyto transient could not be detected in 13 out of 15 measurements ( Fig. 4d , Supplementary Fig. 4a,b , Supplementary Movie 5 ). This indicates a functional link between the second extended [Ca 2+ ] cyto transient and successful fertilization. 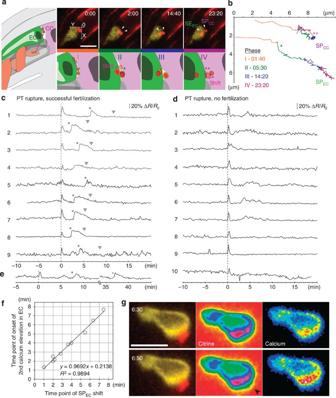Figure 4: A second [Ca2+]cytotransient in egg cells is associated with successful fertilization. (a) Left: scheme depicting SP release from a PT growing around receptive SY (drawn in grey). After burst, SPs are located at the fusion site between EC and CC. Upper panel: time series of LHR SP (red, arrowheads) fertilizing an egg cell expressing the CerTN-L15 sensor (yellow). In the left micrograph, zero and orientation of the coordinate system inbare indicated. Lower panel: scheme of different phases of sperm cell movement before and during fusion. Phase I: parallel movement of sperm cells after arrival along fusion site. Phase II: sideward shift of SPEC(single asterisk) towards EC. Phase III: arrest of SPCCand movement of SPECnucleus towards EC nucleus. Phase IV: sideward shift of SPCC(double asterisk) and subsequent fast sperm nuclei separation. (b) Tracking movement of both sperm cells at fusion site of experiment shown ina. Different colours of the tracks indicate the four different phases and numbers indicate end points of each phase after sperm delivery in minutes. Shift of SPECoccurs at 1:40 min (single asterisk) and shift of SPCCat 14:20 min (double asterisk) in this example. (c) [Ca2+]cytosignals in the EC during successful fertilization. Graphs are normalized and aligned to time of PT rupture (0.0 min). Asterisks mark shift of SPEC, arrowheads mark fast separation of both sperm nuclei indicating successful fertilization of both female gametes. In traces 4 and 5, SPs were not visible at all times. In all cases, two Ca2+transients occur: a short single transient during PT rupture and a longer extended transient after SPECshift (Phase II). (d) Variety of [Ca2+]cytosignals in the EC during unsuccessful fertilization. Only a single Ca2+transient occurs on pollen tube rupture (0.0 min). (e) Exceptional case of EC fertilization. Ratio change of pEC1:CerTN-L15 is shown. SPECdisplays two shifts (asterisk) before fusing with the EC. Each shift is followed by a Ca2+transient in the EC (Corresponding kymograph seeSupplementary Fig. 4d). (f) Correlation of SPECshift towards EC and beginning of second Ca2+transient in EC (n=10). Formula of linear regression and calculated coefficient of determination (R2) are given. (g) Diffusion of sensor molecules into sperm cells upon gamete fusion. Time points before (top row) and after SPECshift (bottom row). Left column, fluorescent micrographs of egg cell (yellow, citrine signal of CerTN-L15) and LHR sperm cell nuclei (red). Middle column, false colour representation of egg cell citrine signal. The dotted line displays the egg cell outline before the SPECshift. The arrowhead indicates spreading of citrine signal towards the position of sperm cells. Scale bars, 20 μm. Figure 4: A second [Ca 2+ ] cyto transient in egg cells is associated with successful fertilization. ( a ) Left: scheme depicting SP release from a PT growing around receptive SY (drawn in grey). After burst, SPs are located at the fusion site between EC and CC. Upper panel: time series of LHR SP (red, arrowheads) fertilizing an egg cell expressing the CerTN-L15 sensor (yellow). In the left micrograph, zero and orientation of the coordinate system in b are indicated. Lower panel: scheme of different phases of sperm cell movement before and during fusion. Phase I: parallel movement of sperm cells after arrival along fusion site. Phase II: sideward shift of SP EC (single asterisk) towards EC. Phase III: arrest of SP CC and movement of SP EC nucleus towards EC nucleus. Phase IV: sideward shift of SP CC (double asterisk) and subsequent fast sperm nuclei separation. ( b ) Tracking movement of both sperm cells at fusion site of experiment shown in a . Different colours of the tracks indicate the four different phases and numbers indicate end points of each phase after sperm delivery in minutes. Shift of SP EC occurs at 1:40 min (single asterisk) and shift of SP CC at 14:20 min (double asterisk) in this example. ( c ) [Ca 2+ ] cyto signals in the EC during successful fertilization. Graphs are normalized and aligned to time of PT rupture (0.0 min). Asterisks mark shift of SP EC , arrowheads mark fast separation of both sperm nuclei indicating successful fertilization of both female gametes. In traces 4 and 5, SPs were not visible at all times. In all cases, two Ca 2+ transients occur: a short single transient during PT rupture and a longer extended transient after SP EC shift (Phase II). ( d ) Variety of [Ca 2+ ] cyto signals in the EC during unsuccessful fertilization. Only a single Ca 2+ transient occurs on pollen tube rupture (0.0 min). ( e ) Exceptional case of EC fertilization. Ratio change of pEC1:CerTN-L15 is shown. SP EC displays two shifts (asterisk) before fusing with the EC. Each shift is followed by a Ca 2+ transient in the EC (Corresponding kymograph see Supplementary Fig. 4d ). ( f ) Correlation of SP EC shift towards EC and beginning of second Ca 2+ transient in EC ( n =10). Formula of linear regression and calculated coefficient of determination ( R 2 ) are given. ( g ) Diffusion of sensor molecules into sperm cells upon gamete fusion. Time points before (top row) and after SP EC shift (bottom row). Left column, fluorescent micrographs of egg cell (yellow, citrine signal of CerTN-L15) and LHR sperm cell nuclei (red). Middle column, false colour representation of egg cell citrine signal. The dotted line displays the egg cell outline before the SP EC shift. The arrowhead indicates spreading of citrine signal towards the position of sperm cells. Scale bars, 20 μm. Full size image Egg cell-specific calcium signature during plasmogamy To reveal the role of the second [Ca 2+ ] cyto transient for plasmogamy, we analysed the timing of associated events in more detail. In animal oocytes, a [Ca 2+ ] cyto elevation occurs after the sperm–egg fusion. In plants, two female gametes are fertilized by two sperm cells. This double fertilization event is supposed to require molecular events such as cell–cell recognition, gamete attachment, sperm cell separation, gamete membrane fusion, egg activation and cell wall modifications that take place between both male–female gamete pairs. Any of these processes may involve calcium signalling. While it is challenging to directly address each process separately, the timing of events before fertilization can be dissected by using a marker line that labels sperm nuclei and tracking their movement at the fusion site [11] . Since both sperm cells do not possess any propelling mechanism, their movement presumably results from elastic deformations and pressure exerted by neighbouring cells or differential surface interactions. Hamamura et al. [11] reported that sperm delivery is composed of three steps. They are delivered as a pair (i) and after a period of immobility lasting about 7.4 min (ii) they both fuse almost simultaneously about 8.5 min after release with either female gamete without any preference (iii). To correlate the second [Ca 2+ ] cyto transient with stages of sperm delivery and fusion, we tracked the sperm nuclei after pollen tube rupture and analysed their trajectories for consistent movement patterns. The sperm cell, which eventually fused with the egg cell, was termed SP EC , while the sperm cell that would fuse with the central cell was termed SP CC ( Fig. 4a ). After pollen tube rupture, we observed four distinct phases of sperm movement, which typically occurred over a travelled distance of 10 μm ( Fig. 4b ): after delivery, both cells moved initially quickly together along parallel trajectories (phase I, Fig. 4b , orange trajectories); a second phase is initiated by a sudden sideward movement of SP EC apart from SP CC ( Fig. 4a,b , single asterisks) followed by slow movement, rotation and temporary arrest (phase II, Fig. 4b , green), while SP CC movement was also slowed down (phase III, Fig. 4b , blue); after a second sudden positional shift, now of SP CC ( Fig. 4a,b , double asterisks), both separated sperm nuclei then made final movements inside the female gametes (phase IV, Fig. 4b , violet) indicating fertilization success. Plotting the intensities of each SP in an overlaying kymograph visualizes their velocity over time ( Supplementary Fig. 4c ). After the arrival of both cells ( t =0), an initial rapid parallel movement (orange phase), followed by a slow down and the eventual separation due to backwards movement of SP CC is visualized. The occurrence of both shifts of SP EC and SP CC in opposite directions is clearly visible in all successful fertilization attempts ( n =10) but absent when fertilization failed ( n =13). The shifts were also observed in both failed fertilization attempts where the second broader [Ca 2+ ] cyto transient was detected but the sperm nucleus did not continue to move towards the nucleus of the female gamete (data not shown). In a single measurement, where delayed or incomplete plasmogamy was observed, we could detect two broader [Ca 2+ ] cyto transients in the egg cell and also two sudden shifts of SP EC ( Fig. 4e , Supplementary Fig. 4d ). These exceptions indicate that the shift can occur repeatedly and therefore could precede successful gamete fusion, eventually representing the event of initial sperm cell adhesion to the female gamete before fusion occurs. To correlate the [Ca 2+ ] cyto signatures in egg cells and the sperm cell movement patterns, we further analysed the occurrence and timing in all measurements where both events could be unequivocally detected ( n =10). We found that the sudden movement of SP EC at the end of sperm movement phase (i) generally coincided with the onset of the second broader [Ca 2+ ] cyto transient ( R 2 = 0.9894; time difference between shift and onset of [Ca 2+ ] cyto transient was 5±13 s; Fig. 4f , Supplementary Movie 4 ). We interpret this finding as strong evidence for a functional link between gamete interaction, Ca 2+ signalling in the egg cell and successful plasmogamy. To determine the time point of plasmogamy as precise as possible, we therefore followed the rational that upon fusion of the plasma membranes of both gametes, cytosolic calcium sensor molecules would immediately diffuse into the sperm cell cytoplasm resulting in detectable citrine fluorescence around the sperm cell nucleus. In four measurements of successful fertilization, measurements were possible as egg cell and SP EC were positioned in the focus plane such that both the fluorescent signals overlapped only minimally. In all four experiments, we were able to detect the spreading of citrine fluorescence signal from the egg cell towards the direction of the sperm cell position immedeately after the SP EC shift, coinciding with the broader [Ca 2+ ] cyto transient ( Fig. 4g , Supplementary Fig. 5 ). In summary, this observation indicates that all three processes, sperm cell shift, onset of the broad [Ca 2+ ] cyto transient and gamete fusion occur all in concert and within less than 20 s. Innovations in specimen handling and application of a sensitive calcium reporter have allowed live-cell observations and detection of cell-type-specific Ca 2+ signatures during the entire double fertilization process in the model plant Arabidopsis . Measuring [Ca 2+ ] cyto in vivo in the female gametophyte at high resolution was previously hampered due to the low accessibility of the deeply embedded cells for imaging. We have optimized a previously reported semi- in vivo fertilization assay that allows live-cell observations by using excised ovules and semi -in vitro grown pollen tubes [32] . Adaptation of this system for confocal fluorescence imaging and expression of sensors driven by cell-specific promoters resulted in reduced background and improved sensitivity. We decided to use the troponin C-based sensor CerTN-L15 as it is expected to be less affected by or interfering with cellular processes as it is the case for calmodulin-based sensors [31] . The improved brightness and high sensitivity of this sensor also present significant advantages for imaging through several cell layers [31] , [39] , [40] and thus enabled us to record changes in [Ca 2+ ] cyto inside the ovule at subcellular resolution. The described experimental setup allowed studies yielding strong evidence for a functional role of Ca 2+ signalling during virtually all steps of the double fertilization process in angiosperms. We were able to confirm recently reported [Ca 2+ ] cyto oscillations in synergid cells during pollen tube interaction [20] and provide further insights into cell–cell communication between these cells and the provoked [Ca 2+ ] cyto transients. One open question was, for example, whether the communication between the pollen tube tip and synergid cells occurs already at a distance as concluded earlier [20] or whether direct cell–cell contact is required. Our measurements show that irregular [Ca 2+ ] cyto elevations can occur spontaneously in synergid cells at a low likelihood, but do not cause cell death. In addition, we observed that only pollen tubes that successfully enter the ovule and interact with the synergid cells induce high persistent [Ca 2+ ] cyto oscillations that may ultimately trigger synergid cell death and pollen tube burst. Usage of a novel marker for the pollen plasma membrane further indicated that physical contact of the pollen tube apex was necessary to induce and maintain [Ca 2+ ] cyto oscillations only in the synergid cell, which was in direct contact with the tube apex. Recently components of the FERONIA (FER) signalling pathway were shown to be involved in the initiation of calcium oscillations and for coupling these with programmed cell death [41] . Stimulus-induced [Ca 2+ ] cyto oscillations have been frequently observed in plants. It was reported that their period, amplitude and waveform encode information about stimulus and trigger required to activate specific signalling responses, to regulate protein activity and eventually to alter gene expression [42] . The spiking nature of the synergid transients is typical for rapidly released Ca 2+ from intra- or extracellular stores followed by slower removal [43] . Observations of comparable [Ca 2+ ] cyto spiking signatures in legume root hairs, for example, induced by symbiotic infection with rhizobial bacteria or mycorrhizal fungi, identified the origin of the [Ca 2+ ] cyto wave at the cell nucleus [44] , [45] , [46] and therefore depend on specific metabotropic receptors at the plasma membrane that perceive and convey the extracellular signal [47] . In contrast, during physical stimulation of root epidermal cells, observed [Ca 2+ ] cyto transients originated from the site of stimulation at the cell periphery [48] , suggesting extracellular stores or peripheral ER as sources of Ca 2+ and possibly the involvement of stretch-activated calcium channels [49] . The localized transients of [Ca 2+ ] cyto in synergid cells also occur in immediate proximity to the cell contact site, which is reminiscent of mechano-sensing. The oscillation signature, however, is similar to that observed during symbiotic infections and thus suggests an involvement of metabotropic receptors and the existence of feedback mechanisms of Ca 2+ -induced Ca 2+ release [50] . The regulation of such oscillatory increases of [Ca 2+ ] cyto commonly occurs through the receptor-mediated activation of phospholipase C, which increases the levels of inositol-1,4,5-trisphosphate (InsP3) that further triggers InsP3-receptor-mediated Ca 2+ release from internal storages. The signalling cascades that might be provoked by [Ca 2+ ] cyto increase in the synergid cells are currently unknown. During self-incompatibility in poppy, it was shown that [Ca 2+ ] cyto increase is correlated with the generation of reactive oxygen species and NO signalling resulting in cell death. Downstream targets include, for example, components of the cytoskeleton and mitogen-activated protein kinases [51] . Both synergid cells undergo cell death either during pollen perception or after successful fertilization [52] , [53] . We observed that only synergid cells showing high and continuous amplitudes burst during pollen tube interaction. This finding supports previous reports also in animal cells showing that high sustained [Ca 2+ ] cyto levels are toxic to cells and may result in cell death both during necrosis and apoptosis [54] . The identification and analysis of calcium-dependent signalling components in synergid cells will now be an exciting area of future research activities. Reactive oxygen species were recently reported to mediate pollen tube burst in [Ca 2+ ] cyto -dependent processes [55] suggesting the existence of similar mechanisms during synergid cell death. It will be of similar importance to identify the pollen tube apex-derived stimulus and synergid cell surface receptors involved in triggering the described [Ca 2+ ] cyto oscillations. Our results on [Ca 2+ ] cyto oscillations support the notion of a short-range signal secreted from the pollen tube apex that is perceived by receptor(s) of synergid cells triggering a feedback mechanism that cause localized, oscillating release of Ca 2+ . The FERONIA receptor-like kinase and the glycosylphosphatidylinositol-anchored LORELEI protein are candidate synergid cell surface proteins that have previously been shown to be required for pollen tube burst [6] , [7] . Moreover, a secreted peptide, RALF (rapid alkalinization factor) was recently shown to activate FERONIA in the root [56] . Whether RALF peptides secreted from the pollen tube apex activate FERONIA at the surface of synergid cells inducing [Ca 2+ ] cyto oscillations remains to be determined. Further studies should also involve mutants with defects in phospholipase C/InsP3 signalling and metabotropic receptors (see above). Altogether, these mutants will be instrumental in elucidating the functional importance of the localized [Ca 2+ ] cyto oscillations in the synergid–pollen tube interaction. During the next act of plant double fertilization, the fusion of sperm cells with both female gametes, an involvement of Ca 2+ transients was long suggested by pioneering work applying in vitro fertilization studies with maize egg and sperm cells [23] , [24] , [25] . It was reported that Ca 2+ influx occurred after egg–sperm fusion and spreads as a wave front from the fusion site towards the whole cell. However, these studies did not allow to image [Ca 2+ ] cyto dynamics during the whole fertilization process and thus overlooked, for example, the first [Ca 2+ ] cyto transient in both female gametes that is correlated with sperm cell release. The function of this first elevation remains unclear. It might also be correlated with mechanic deformation of female gametes, albeit we did not observe [Ca 2+ ] cyto transients in egg cells, which were occasionally deformed by pollen tubes (see above). It was, however, recently shown that egg cells secrete EC1 protein after pollen tube burst to activate sperm cells and thus enable them to fertilize female gametes [12] . Thus, the egg cell itself requires activation shortly after the sperm cell release. Further studies will elucidate whether egg activation at this phase requires Ca 2+ signalling. Mammalian egg cells are activated by a series of [Ca 2+ ] cyto oscillations that occur shortly after egg–sperm membrane fusion (for review, see ref. 57 ), thus differing significantly from the single elevation that we have observed during pollen tube burst. A major difference between previously reported in vitro and our semi -in vivo studies is the length of [Ca 2+ ] cyto elevations. It was reported that the [Ca 2+ ] cyto transient after in vitro gamete fusion lasted for up to 30 min, while we observed that the comparable second extended [Ca 2+ ] cyto transient lasted on average only for 3 min. Moreover, the signature of this [Ca 2+ ] cyto transient is different and seems to consists of a few very short spikes, which could not be resolved individually. In agreement with the above-mentioned in vitro studies, we conclude that this [Ca 2+ ] cyto transient was provoked by fusion rather than adhesion. A functional role of the reported Ca 2+ influx could not be addressed during in vitro studies. We were able to ultimately correlate the second [Ca 2+ ] cyto transient with plasmogamy and fertilization success. In a parallel study, Hamamura et al. [58] found highly similar [Ca 2+ ] cyto signatures during egg cell fertilization using the calcium sensor YC3.60. In line with our findings, the authors also identified a correlation between the occurrence of the second [Ca 2+ ] cyto transient and successful fertilization. In a mutant of the HAP2/GCS1 gene, which has known roles in pollen tube guidance and fertilization, sperm cells were delivered properly but gamete fusion never occurred. Consistently, the authors found that in this mutant the second [Ca 2+ ] cyto transient in the egg cell was not detectable. It will, however, remain challenging to elucidate the exact role of Ca 2+ –dependent signalling during this short fertilization phase. In mammals, two separate fusion phases are distinguished after gamete adhesion takes place: a marginal and a separating phase [59] . During the marginal phase, fusion is initiated and the second phase, which has a different topological character, fusion is completed during a process similar to endocytosis. We suggest that this process is similar in plants. In accordance with the topology of the marginal phase, we observed egg cell cytoplasm extending towards the sperm cell followed by a quick shift of the sperm cell towards the inside of the egg, which might be consistent with the separating phase characterized by endocytosis at the plasma membrane. Moreover, we have observed few cases that showed additional [Ca 2+ ] cyto elevations displaying the signature of the extended second transient. We assume that fusion was initiated in these cases, but not completed allowing additional fusion events associated with [Ca 2+ ] cyto transients. Markers labelling the plasma membrane and cytoskeleton of gametes in combination with Ca 2+ sensors whose signals can be optically separated from the gamete surface will help to explain these observations. While diffraction-limited confocal imaging of fertilization presents a significant advance, unequivocal visualization of membrane fusion may also require substantially improved spatial resolution. It also remains to be determined which downstream responses are triggered by these relatively short [Ca 2+ ] cyto transients. It is very likely that the structure of the cytoskeleton undergoes local changes and reorganization to initiate the first fusion phase and to enable the transport of the sperm nucleus towards the egg nucleus. It was also discussed that [Ca 2+ ] cyto transients initiate the formation of cell wall material after fusion likely representing a block to polyspermy functionally similar to the fertilization membrane in animals [24] . In animal oocytes, [Ca 2+ ] cyto waves triggered by fusion with the first sperm elicit immediate exocytosis of extracellular matrix-modifying enzymes to quickly block polyspermy [15] . In vitro fertilization studies in maize showed the formation of cell wall components already 30 s after gamete fusion [60] indicating a quick release of cell wall components likely from trans-golgi vesicles stored in the egg cell. Whether this leads to a block of polyspermy, whether it also occurs in vivo and depends on Ca 2+ signalling remains to be determined. However, the timing and the observation that central cell fusion lacks the second [Ca 2+ ] cyto transient and allows polyspermy [61] suggest that the egg cell-specific [Ca 2+ ] cyto transient might also be involved to generate a quick block to polyspermy. In vitro fertilization studies using egg and central cells of tobacco confirm our finding that the second transient Ca 2+ elevation is lacking in central cells [62] . In conclusion, we have reported [Ca 2+ ] cyto dynamics during the entire double fertilization process and were able to correlate the timing of Ca 2+ signatures with cellular events including localized cross-talk between the pollen tube apex and synergid cells, pollen tube burst and sperm delivery, as well as gamete activation and fusion culminating in fertilization success and likely a polyspermy block to the egg cell. These studies thus significantly extend our knowledge about the timing of double fertilization events and deepen our understanding about the role of Ca 2+ signalling during the individual processes. Future studies are necessary to unveil the molecular players involved in [Ca 2+ ] cyto induction, signal maintenance and/or oscillation as well as the downstream targets regulating Ca 2+ dependent processes to finally understand its role during double fertilization. Generation of CerTN-L15 expressing plants The coding sequence of CerTN-L15 (ref. 31 ) was amplified using the primers P12 (5′-GGGGACAAGTTTGTACAAAAAAGCAGGCTGCCACCATG-3′) and P16 (5′-GGGGACCACTTTGTACAAGAAAGCTGGGTTCA-3′). The resulting PCR product was used in a BP-reaction (Gateway Technology manual; Life Technologies) with the donor vector pDONR207 (Invitrogen) resulting in pDONR207-CerTN-L15. Sac I/ Spe I restriction digest was performed to remove the 35S promoter of the destination vectors pB2GW7 and pH2GW7 (ref. 63 ), respectively, which was subsequently replaced by the promoters of either AtEC1.1 (ref. 12 ) (454 bp upstream of the start codon of At1g76750), AtMYB98 (ref. 33 ) (1.494 bp upstream of the start codon of At4g18770) or AtDD65 (ref. 34 ) (1.246 bp upstream of the start codon of At3g10890). The EC1.1 promoter was amplified using the primers P9 (5′-CAAAAGCTG GAGCTC TCTAGAG-3′) and P10 (5′-GGCCG ACTAGT ATCCTTCTCAAC-3′) from the plasmid pEC1.1-GUS [12] . The promoter pMYB98 was amplified with the primers P7 (5′-ATG GAGCTC GCGTCGACAGTTG-3′) and P8 (5′-AGGGACTG ACTAGT GGATC-3′) from the plasmid pN7-Myb-EC1 (S. Sprunck, unpublished). pDD65 was amplified using the primers pDD65_FW (5′-AGT GAGCTC AATCAAAATTTAACATTTAAATAAAGTC-3′) and pDD65_REV (5′-TGATT ACTAGT ATCCTTTTCTACTTTGTTTTTGTTTTTGTGCT-3′) from Arabidopsis Col-0 genomic DNA ( Sac I and Spe I restriction sites underlined in primer sequences). CerTN-L15 (pDONR207-CerTN-L15) was recombined into the four destination vectors pB2GW7, pB2GW7-pEC1, pB2GW7-pMYB98 and pH2GW7-pDD65 by LR reaction (Gateway technology, Life Technologies) according to the manufacturer’s protocol. Resulting expression constructs (p35S::CerTN-L15, pEC1::CerTN-L15, pMYB98::CerTN-L15 and pDD65::CerTN-L15) were transformed into Arabidopsis Col-0 plants by floral dipping [64] . Transformants were selected according to their selection marker and fluorescent properties. Generation of the double marker line LHR The promoter pLat52 was amplified from Lat52::GFP expressing plants [65] using the primers FV01 (5′-gggg gagctc ATACTCGACTCAGAAGGTATTGAGG-3′) and FV02 (5′-gggg actagt tttaaattggaatttttttttttgg-3′) and cloned into the destination vector pB2GW7 (ref. 63 ) by replacing the 35S promoter using the introduced SacI and a SpeI sites, resulting in the destination vector pVOLat52GW. TagRFP was amplified from pTagRFP-C (Evrogen) with the primers ptagRFPfwd (5′-caccatggtgtctaagggcgaagagctg-3′) and ptagRFPrev (5′-tggctgattatgatcagttatctagatcc-3′) followed by insertion into the pENTR/D-TOPO vector according to the manufacturer’s protocol (Gateway Technology manual; Life Technologies) to obtain pENTR-tagRFP. To yield pENTR-tagRFP-T, site-directed mutagenesis was performed (QuikChange II Site-Directed Mutagenesis Kit, Agilent) using the primers tagRFP-TPOINT (5′-CTGGAAGGCAGAACCGACATGGCCCTG-3′) and TagRFP-TPOINTrev (5′-CAGGGCCATGTCGGTTCTGCCTTCCAG-3′). A C-terminal 109 nucleotide sequence of MtSYMREM1 (ref. 66 ), covering the C-terminal remorin anchor, was amplified from pDONR207-MtSYMREM1 with the primers FV03 (5′-GGG GAATTC TGGGGAAGAAATCCTCAAGGTAGAG-3′) and FV04 (5′-CCCC GGATCC CTAACTGAAAAACCTTAAACCGCTG-3′). The resulting PCR product was cloned into pENTR-tagRFP-T using the introduced EcoRI and BamHI restriction sites (underlined) to obtain pENTR-tagRFP-T-REM. The expression construct pP Lat52 :tagRFP-T-REM was created by LR reaction (Gateway Technology, Life Technologies) with pENTR-tagRFP-T-REM and pVOLat52GW. To create the double marker line Lat52:tagRFP-T-REM; HTR10:HTR10-mRFP (LHR), pP Lat52 :tagRFP-T-REM was used to transform plants homozygous for HTR10:HTR10-mRFP [38] by floral dipping [64] . Transformants were selected according to their selection marker and fluorescent properties. Growth conditions of Arabidopsis thaliana Arabidopsis plants were either grown under short day conditions (8 h light, 20 °C, 50–70% relative humidity) for 4–6 weeks followed by long day conditions (16 h light, 20 °C, 50–70% relative humidity) or continuously grown under long day conditions. Root imaging Roots were prepared for imaging using the RootChip, a microfluidic perfusion device as described previously [35] , [67] . In brief, seeds were sterilized, placed on cut pipet tips (5 mm) that were filled with MS medium [68] and incubated for 4 days under long day conditions in a growth chamber (16 h, 20 °C, 50–70% relative humidity). Seedlings were transferred to the RootChip and incubated for one additional day in liquid MS medium. Images were acquired every 3 s. Growing roots were continuously perfused with ½ strength MS medium and treated with square pulses of 200 m M mannitol over 5 min. Semi- in vivo pollen tube growth assay Semi- in vivo experiments were performed with modifications from the originally described assay [32] using modified pollen germination medium (PGM) [69] containing 18% sucrose, 0.01% boric acid, 1 m M MgSO 4 , 1 m M CaCl 2 , 1 m M Ca(NO 3 ) 2 , 5 m M MES and 0.75% ultrapure agar (Version 1) or 0.175% agarose (peqGold Universal) (Version 2). The pH was adjusted to 7.0 with 200 m M KOH. The pistils and ovules that were used in all experiments were dissected from flowers with not yet opened anthers to ensure that only pollen used for pollination will fertilize the observed ovules. Preparation of pistils was performed by removing the leaves and anthers from the flower with forceps (Dumont No. 5) followed by cutting the pistil at junction of style and ovary with a razorblade and placing it upright on solidified PGM. Pollen was used from freshly opened anthers and put directly on the stigma of the cut pistils. For dissection of ovules, a pistil was cut open at the replum with the tip of a 27-gauge needle and the ovules were removed from the placenta using the needle. All dissections were performed on a microscope slide with double-sided tape to fix the tissue, but the contact of all tissue parts used for the assay with the adhesive tape was avoided. Modified semi- in vivo assay Version 1: A round plastic chamber (Ø1 × 1 cm), which was covered and sealed on one side with a microscope slide, was completely filled with 1 ml fresh PGM containing 0.75% agar. Medium was solidified for 30 min. The pollinated pistils and the individual ovules were placed on the medium surface. Afterwards, the chamber was covered by a cover slip with spacers of modelling clay, in a way that an air cushion was created between specimen and cover glass. The chamber was incubated at room temperature with light for 3 to 5 h. When the pollen tubes left the cut pistil and grew towards the dissected ovules, the chamber was turned cover glass-side down, the microscope slide was removed and the air cushion was released slowly, by puncturing the modelling clay with a needle. Thus, the agar helped to immobilize the tissue at the cover slip without disturbing the arrangement of the pistil and the ovules. After an additional incubation for 30 min, the chamber was used for imaging. Version 2: All preparations were done under humidified conditions with a relative humidity of >80% by dissecting under a hood containing a humidifier. Pistils were cut and placed vertically on solid PGM containing 0.75% (w/v) agar. Stigmas of the pistils were pollinated and incubated for 3 h in the humidified chamber with light. Just before pollen tubes emerged from the pistil (usually ~3.5 h after pollination), pistils were transferred into a two-well microscope μSlide (IBIDI) that was filled with half solid PGM containing 0.175% (w/v) agarose. Before filling the μSlide with PGM, a 0.5-mm thick silicon mat with small slots, cut in the centre of the silicon layer, was placed on the bottom of the μSlide wells. Pistils were carefully pushed through the PGM to the bottom of the slide and fixed horizontally in the edges of the slots in the silicon layer. Afterwards, the ovules were dissected and transferred to the μSlide. They were pushed through the PGM with thin glass needles, pulled with a micropipette puller (P-97, Sutter Instruments), and placed in front of the cut pistils. The slides were covered with a lid and incubated in the humidified chamber with light. When pollen tubes had reached the ovules the μSlide was transferred to the microscope for imaging. Microscopy Imaging of the RootChip experiments was performed on an inverted epifluorescence microscope (LeicaDMIRE2) using a × 10 objective (Leica, 0.40 N.A., Air). For excitation of the sensor, a Polychrome V monochromator light source (TILL Photonics, Germany) was used. Fluorescence signals were detected using a Dual View beam splitter (Photometrics, USA) containing an ET470/24 m and ET535/30m filter setup and an EMCCD camera (QuantEM:512SC; Photometrics). Semi- in vivo experiments were either done on an inverted Leica DMI6000B microscope using a × 40 objective (Leica, 1.25 N.A., Oil) equipped with a Yokogawa (Japan) CSU-X spinning disk confocal head and a motorized stage (ASI, USA) for automated multiposition imaging or on a Leica SP8 inverted confocal laser scanning microscope using a × 40 objective (Leica, 1.3 N.A, oil). Using the Leica DMI6000B microscope, fluorophores were excited at a wavelength of 441 nm (Cerulean), 514 nm (Citrine) and 561 (RFP/tagRFP) using a multiband dichroic mirror (445/515/561 nm dichroic beamsplitter, Semrock, USA) and the fluorescence signal was detected with an Evolve EMCCD camera (Photometrics, USA) using band-pass emission filters (475/42, 540/15 narrow, 605/64 RFP, Semrock). Exposure times were 100 ms (Citrine), 300 ms (Cerulean) and 600 ms (RFP). Acquisition was controlled using SlideBook 5.0 software (Intelligent Imaging Innovations, USA). Using the Leica SP8, fluorophores were excited with the same wavelengths described for the spinning disk system. Emission was detected using band-pass filter settings (Cerulean: 462–510 nm; Citrine: 520–550 nm and RFP/tagRFP: 570–666 nm). Image processing and data analysis Image processing and analysis were performed using FIJI ( http://fiji.sc/ ). To correct for movements or growth, images were registered using the StackReg plug-in ( http://bigwww.epfl.ch/thevenaz/stackreg/ ). To create false colour ratiometric images for FRET experiments, the RatioPlus plug-in ( http://rsbweb.nih.gov/ij/plugins/ratio-plus.html ) and a 16-colour lookup table were used. For false colour ratiometric images as shown in Fig. 1b , raw data were processed as follows: multiplication of both ‘FRET’ channels (acceptor emission under donor excitation) with the reference channel (acceptor emission under acceptor excitation), 32-bit conversion, application of a mean filter with a radius of five pixels to both images, thresholding (Otsu-method) over the stack histogram. Dividing the acceptor channel by donor channel resulted in the ratiometric image (16-colour lookup table). Analysis of FRET ratio changes was performed by calculating the ratio of fluorescence intensities of acceptor and donor under donor excitation using the MultiMeasure plug-in ( http://www.optinav.com/imagej.html ) in specific regions of interest ( Supplementary Fig. 6 ). The regions were 50 × 50 μm in root experiments and 4 × 4 μm squares for subcellular analysis or polygons in shape of the synergid cells for single cell analysis. The values of those measurements were further analysed in Excel. The ratios of acceptor and donor were normalized ((Ratio[ t ]−Ratio[ t 0 ])/Ratio[ t 0 ]) to display the relative ratio change over time. For the analysis of the [Ca 2+ ] cyto oscillation in synergids, the individual 4 × 4 μm regions were aligned as described ( Fig. 2d ) and the regions were moved over time, following the position of the growing pollen tube tip. The amplitudes of the ratio changes in individual regions were calculated and the amplitude values of one oscillation event were normalized to the amplitude in region D1/L1. To define significant [Ca 2+ ] cyto oscillations in synergid cells, a base line was determined as the mean ratio change over 10 min of FRET measurement before a pollen tube was in contact with the synergid cell. To determine the significance of amplitudes, the traces were smoothened applying a sliding average of three time points, the first derivative was calculated and the s.d. of the baseline (30 min without cell–cell interaction) of the resulting curve was determined. Amplitudes exceeding the s.d. of the baseline by fivefold (5 × σ ) were considered significant. Tracking of sperm cells was performed with the FIJI TrackMate plug-in ( http://fiji.sc/TrackMate ) and resulting coordinates were plotted using excel. Kymographs for the analysis of sperm cell movement at the gamete fusion site were generated using the MultipleKymograph plug-in ( http://www.embl.de/eamnet/html/body_kymograph.html ) along a segmented line that covered the track of each sperm cell separately. To compare the movement speed of the two sperm cells, the individual Kymographs were aligned with the starting point of the sperm cell movement overlaying with each other. How to cite this article : Denninger, P. et al. Male–female communication triggers calcium signatures during fertilization in Arabidopsis . Nat. Commun. 5:4645 doi: 10.1038/ncomms5645 (2014).